Competing ordered states with filling factor two in bilayer graphene The quantum Hall effect, in which a two-dimensional sample’s Hall conductivities become quantized, is a remarkable transport anomaly commonly observed at strong magnetic fields. However, it may also appear at zero magnetic field if time-reversal symmetry is broken. Charge-neutral bilayer graphene is unstable to a variety of competing and closely related broken symmetry states, some of which have non-zero quantized Hall conductivities. Here we explore those states by stabilizing them with external fields. Transport spectroscopy measurements reveal two distinct states that have two quantum units of Hall conductivity, stabilized by large magnetic and electric fields, respectively. The majority spins of both phases form a quantum anomalous Hall state, and the minority spins constitute a Kekulé state with spontaneous valley coherence for phase I and a quantum valley Hall state for phase II. Our results shed light on the rich set of competing ordered states in bilayer graphene. Because of its large density-of-states and the 2π Berry phase near its low-energy band-contact points [1] , [2] , [3] , [4] , [5] , [6] , neutral bilayer graphene (BLG) at zero magnetic field ( B ) is susceptible to chiral-symmetry breaking, leading to several gapped spontaneous quantum Hall (QH) states distinguished by valley- and spin-dependent quantized Hall conductivities [7] , [8] , [9] , [10] , [11] , [12] , [13] , [14] , [15] , [16] , [17] , [18] , [19] , [20] , [21] , [22] , [23] , [24] , [25] , [26] , [27] , [28] , [29] , [30] , [31] , [32] , [33] , [34] . In these states, each spin-valley flavour spontaneously transfers charge between layers [10] , [11] . When spin is ignored, only two classes of gapped states can be distinguished: (i) ones in which electrons in opposite valleys are polarized to opposite layers, producing a quantum anomalous Hall (QAH) state with broken time-reversal symmetry and orbital magnetization [7] , [8] , [9] , and (ii) states in which electrons in opposite valleys are polarized to the same layer, yielding a quantum valley Hall (QVH) state with broken inversion symmetry and Hall conductivity, σ H =0 (refs 7 , 8 , 9 ). For spinful electrons, symmetry-broken states further include the layer antiferromagnetic state (LAF) and the quantum spin Hall state with two-terminal conductivity 0 and 4 e 2 / h , respectively. An additional competing state is the Kekulé order with spontaneous coherence between valleys. 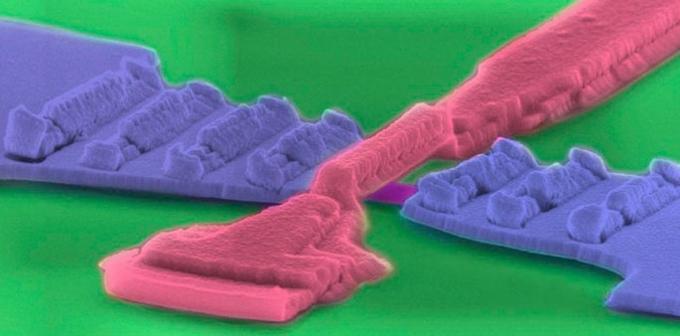Figure 1: SEM image of a dual-gated device. False colored SEM image of a device with suspended bilayer graphene (deep pink), clamped on by source-drain electrodes (cobalt blue) and straddled from above by a suspended top gate (bright pink). Electronic configurations of these states are summarized in Table 1 . Table 1 Schematic diagram of electronic configurations of the states stabilized by electric field and magnetic field. Full size table So far, only the LAF state, which has QVH states with opposite layer polarization signs for opposite spins [8] and appears to be the thermodynamic ground state [35] , [36] , [37] , and (at finite interlayer electric field E ⊥ ) the layer polarized state, which has QVH states with spin-independent layer polarization, have been observed experimentally [35] , [36] , [37] , [38] . Other spontaneous QH states, and competing states with Kekulé order, have eluded experimental observation (although prior work on singly gated devices has shown that the QH states at filling factors ν =4 and ν =0 can persist to very small B [39] ). The experiments we describe are motivated by the sensitivity of the competing orders in BLG to both E ⊥ and B fields. Spontaneous Hall states can be explored by taking advantage of their adiabatic connection to QH states at integer filling factors within BLG’s eightfold degenerate lowest Landau levels (LLs). Our prior work [40] has shown that the LL gaps in dual-gated devices with controlled layer polarization are different from those in singly gated devices. Here we use transport spectroscopy [35] , [36] , [40] to study high-quality dual-gated suspended BLG devices at ν =±2 (refs 36 , 38 , 39 , 41 , 42 , 43 , 44 , 45 , 46 ) as a function of B and E ⊥ . Our results reveal two distinct states: (1) phase I is fully resolved only near E ⊥ =0 and large B , and has a relatively small gap that extrapolates to 0 at B =0. This phase is expected [8] to be spontaneously spin-polarized and to have coherence between valleys (layers), that is, with Kekulé valley order [47] , [48] , [49] , (2) phase II appears only at finite E ⊥ , but can be stabilized at a much smaller B and has a much larger gap with a finite B =0 intercept, suggesting that this state survives to anomalously weak B . Because finite B couples to the spin and orbital moments, and finite E ⊥ favours layer (valley) polarization, this state is expected [8] to form a majority-spin QAH state but a minority-spin QVH state, where majority (minority) spins refer to those that occupy all four (half) of the orbital-degenerated LLs. It follows that its charge, spin and valley Hall conductivities are all quantized to 2 e 2 / h . The anomalous stability of phase II at small B is consistent with the stability of QVH (QAH) state at large E ⊥ (finite B ). Our results represent the first spectroscopic mapping of the exotic behaviour hosted in BLG at filling factor ν= 2. By shedding light on the competition between ordered states in BLG, we provide a road map for studying the spontaneous symmetry breaking in BLG and its thicker chiral cousins [8] , [50] , [51] , [52] . Realization of two distinct ν= ±2 QH states Suspended dual-gated devices ( Fig. 1 ) with mobilities as high as 150,000 cm 2 V −1 s −1 were measured in He-3 refrigerators. Here we present data from two different devices (devices 1 and 2) with field effect mobilities 80,000 and 40,000 cm 2 V −1 s −1 , respectively. (Similar data are observed in two additional devices). All measurements were taken at temperature T =260 mK. Figure 1: SEM image of a dual-gated device. False colored SEM image of a device with suspended bilayer graphene (deep pink), clamped on by source-drain electrodes (cobalt blue) and straddled from above by a suspended top gate (bright pink). 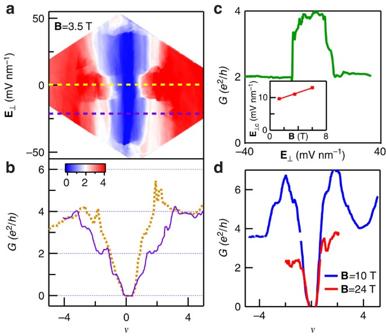Figure 2: Magnetotransport data. (a)G(E⊥, n)of device 1 atB=3.5T. (b) Line tracesG(ν) atB=3.5 T andE⊥=0 (brown dotted line) andE⊥=−21 mV nm−1(purple solid line), respectively. (c) Line traceG(E⊥) atB=3.5 T and filling factorν=2 (densityn=1.7 × 1011cm−2). Data ina–care from device 1. Inset: critical electric fieldEcversusBand linear fit to the data points with slope ~0.72 mV nm−1T−1. (d)G(ν) of device 2 atE⊥=0, andB=10 and 24 T, respectively. Full size image Figure 2a plots the two-terminal differential conductance G of device 1 in units of e 2 / h at B =3.5 T as a function of charge density n and out-of-plane electric field E ⊥ . The QH plateaus at ν= 0, ±1, ±2 and ±4 appear as dark blue, blue, white and red colour bands, respectively. Most interestingly, the resolution of ν= ±2 QH states depends on E ⊥ . This can be seen in the G ( ν ) traces in Fig. 2b , near E ⊥ =0, only the QH plateaus at ν= 0 and ±4 are fully resolved; in contrast, at larger E ⊥ =− 21 mV nm −1 , the ν= ±2 plateaus are clearly visible. The resolution of the ν= ±2 states is abrupt: at ν= 2, G( E ⊥ ) stays at 4 e 2 / h for small E ⊥ , but drops sharply to a 2 e 2 / h plateau at a well-defined critical value E ⊥ c . This critical E ⊥ c is ~10 mV nm −1 at 8 T, and is only weakly dependent on B , with a slope ~0.72 mV nm −1 T −1 ( Fig. 2c ). Figure 2: Magnetotransport data. ( a ) G( E ⊥ , n) of device 1 at B =3.5T. ( b ) Line traces G (ν) at B =3.5 T and E ⊥ =0 (brown dotted line) and E ⊥ =− 21 mV nm −1 (purple solid line), respectively. ( c ) Line trace G ( E ⊥ ) at B =3.5 T and filling factor ν =2 (density n= 1.7 × 10 11 cm −2 ). Data in a – c are from device 1. Inset: critical electric field E c versus B and linear fit to the data points with slope ~0.72 mV nm −1 T −1 . ( d ) G (ν) of device 2 at E ⊥ =0, and B =10 and 24 T, respectively. Full size image The above observations reflect unprecedented sample quality, but agree with previous studies in which the ν= 2 state is fully resolved only when E ⊥ is non-zero either in a controlled fashion in dual-gated devices [36] , [38] , or inadvertently in singly gated devices [35] , [37] , [43] , [45] . This suggests that the ν= 2 state observed at B =3.5 T is layer polarized. The intriguing possibility of a ν= 2 state at E ⊥ =0 in higher quality samples or in stronger fields has not been demonstrated previously. Figure 2d displays G ( ν ) for device 2. As in the case of device 1, for B <20 T, the ν =2 state is resolved only in the presence of finite E ⊥ . At E ⊥ =0, the state is fully resolved for B >24 T. Characterization of the two distinct ν= ±2 QH states The experimental observation presented above allows us to identify the nature of these two distinct ν= 2 QH states. Phase I is only fully resolved at E ⊥ =0 and large B , and phase II is resolved at large E ⊥ and relatively small B . To further explore these two distinct ν= 2 QH states, we perform transport spectroscopy by using the source-drain bias V as a spectroscopic tool [35] , [40] . The details of this measurement technique and its application to QH states can be found in refs 36 , 40 . Briefly, at each conductance plateau, BLG’s Fermi level is pinned between the highest filled and the next unfilled LLs. Charges are carried by edge states that are separated from the gapped bulk by a gap on the order of the LL spacing. Increasing bias aligns the source electrode’s Fermi level with the next unfilled LL and allows additional charge transport through the bulk. Consequently, near V =0, the device displays a conductance valley, whose half-width yields the LL gap Δ . 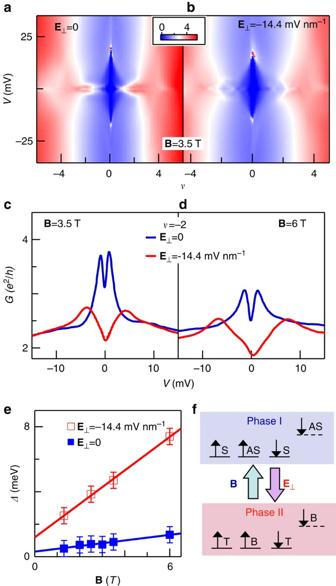Figure 3: Transport spectroscopy data from device 1. (a,b)G(V,n) atE⊥=0 and−14.4 mV nm−1, respectively. Data are taken atB=3.5 T. (c) Line tracesG(V) atν=−2 andB=3.5 T. Blue and red traces are taken atE⊥=0 and−14.4 mV nm−1, respectively. (d) Similar data taken atB=6 T. (e) Measured LL gapΔ(B) atν=2 andE⊥=0 and −14.4 mV nm−1, respectively. Error bars are estimated from bias resolution and uncertainties in the valley width measurement. (f) Schematics of transitions between phases I and II atν=2. (T/B, top/bottom layer; S, symmetric state |S>:=|T>+|B>; |AS>: antisymmetric state |T>−|B>). Figure 3a,b displays G ( V,ν ) from device 1 at B =3.5 T and E ⊥ =0 and −14.4 mV nm −1 , respectively. At E ⊥ =−14.4 mV nm −1 , the diamond at ν=− 2 is significantly larger than that at E ⊥ =0, demonstrating an enlarged LL gap. Such difference in gap sizes can be seen more clearly in line traces in Fig. 3c , which are taken from Fig. 3a,b at ν =−2, respectively. Similar traces at B =6 T are shown in Fig. 3d . At E ⊥ =−14.4 mV nm −1 , prominent zero-bias valleys appear in G ( V ) traces ( Fig. 3c,d , red lines), indicating that the ν =−2 state (phase II) is fully resolved. In contrast, at E ⊥ =0, the G ( V ) traces display only small conductance dips superimposed on a peak at zero bias ( Fig. 3c,d , blue traces), suggesting that phase I is only partially resolved. Figure 3: Transport spectroscopy data from device 1. ( a , b ) G ( V,n ) at E ⊥ =0 and − 14.4 mV nm −1 , respectively. Data are taken at B =3.5 T. ( c ) Line traces G ( V ) at ν =−2 and B =3.5 T. Blue and red traces are taken at E ⊥ =0 and − 14.4 mV nm −1 , respectively. ( d ) Similar data taken at B =6 T. ( e ) Measured LL gap Δ( B ) at ν =2 and E ⊥ =0 and −14.4 mV nm −1 , respectively. Error bars are estimated from bias resolution and uncertainties in the valley width measurement. ( f ) Schematics of transitions between phases I and II at ν= 2. (T/B, top/bottom layer; S, symmetric state |S>:=|T>+|B>; |AS>: antisymmetric state |T>−|B>). Full size image The measured values of Δ ν=−2 are shown in Fig. 3e . At E ⊥ =0, the LL gap for phase I is Δ I ~0.17 meV T −1 with a zero intercept at B =0; in contrast, at E ⊥ =−14.4 mV nm −1 , the gap for phase II is larger by more than a factor of 5, Δ II ~ 1.0 meV T −1 , with a non-vanishing B =0 intercept. We now discuss the nature of these two distinct ν= 2 QH states. Phase I is only fully resolved at E ⊥ =0 and large B , with a vanishing LL gap at B =0. The fact that a large B is required to stabilize this phase has been anticipated in BLG QH ferromagnetism theory [5] , [8] , [22] . In the absence of interactions, the zero-energy LLs are eightfold degenerate and QH effects only exhibit at ν=±4; thus interactions are necessary to induce phase I. Since the valley K and K′ states in the N =0 subspace are localized at the top and bottom layers, respectively, the valley pseudospin and layer pseudospin coincide. At E ⊥ =0, there is an electrostatic energy cost of valley (or equivalently layer) polarization, and it is energetically favourable to achieve a gap at ν= 2 by establishing coherence between the valleys/layers. This is what is observed experimentally: as phase I is only observed in the absence of E ⊥ , it is evidently not layer polarized but a symmetric linear combination of the top and bottom layers. Such a state is also a valley symmetric state, that is, a valley-Kekulé order in the presence of B due to electron–electron interactions. This Kekulé order appears at large B , even though it is absent at B =0. Accordingly, our experiments demonstrate that the stability of the Kekulé state, as measured by its gaps, disappears as B goes to zero. The valley-Kekulé order that we have observed is reminiscent of the Kekulé lattice distortion proposed for carbon nanotubes and graphene [47] , [48] , [49] , albeit here it only exists in the presence of a magnetic field. As B approaches 0, a spontaneous QH state [8] emerges as the ground state, as observed previously [36] . In the absence of B fields, the intervalley interactions in BLG are too weak to induce any valley coherence. At finite B , however, owing to the equivalency of the layer and valley pseudospins, any interlayer coherence naturally leads to intervalley coherence. In contrast to phase I, phase II is observed at anomalously small B and large E ⊥ , with a LL gap that extrapolates to a finite B =0 intercept. Its appearance at much smaller B than phase I is reminiscent of the spontaneous QH states at B =0 (refs 8 , 9 ). This phase is adiabatically connected to the B =0 collinear ferromagnet ordered state with a majority-spin QAH state and a minority-spin QVH state [6] , [8] , [22] . Indeed phase II is only metastable [6] , [8] at B =0, most likely because it loses the ordering competition to the LAF state at E ⊥ =0 and to the QVH state at E ⊥ ≠0. As observed here, however, phase II can be preferred in the presence of finite B and E ⊥ , since states with different total Hall conductivity are most stable at different carrier densities; moreover, the energy of this phase is lowered by the orbital and spin coupling to B and by the compensation of the Hartree energy cost of its layer polarization by E ⊥ . It is partially polarized in spin, valley and layer, and is consistent with a QH ferromagnet state [5] , [8] , [22] , [43] . In terms of their layer characteristics, phase I has XY valley (layer) coherence order, whereas phase II has layer polarization Ising order. Schematic representations of these two phases are provided in Fig. 3f . Here S and AS indicate symmetric and antisymmetric combination of the K and K′ valleys, respectively. The energy differences between these two phases arise mainly from (i) the Hartree energy of layer polarization, and (ii) the difference between interlayer and intralayer exchange for the occupied N =0 LLs. Both differences scale as (d / l β ) × (e 2 / l β ) ~ B , in agreement with the weak linear B dependence of E ⊥ c in our BLG measurements, where the layer separation d is much smaller than the magnetic length l β . We also note that data from singly gated devices are similar to those at finite E ⊥ : owing to the presence of an inadvertently induced electric field ne /2 ε 0 (here ε 0 is the permittivity of vacuum), the ν= ±2 states in singly gated devices are almost always in phase II and stabilized by E ⊥ . Thus, care must be taken when interpreting QH data from singly gated devices. Finally, using transport spectroscopy, we explore the dependence of the LL gap on E ⊥ . 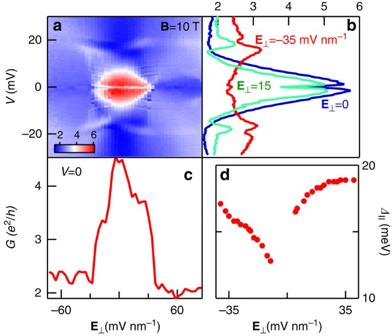Figure 4: Spectroscopy data from device 2 atB=10 T andν=2. (a)G(V,E⊥) data. (b) Line tracesG(V) atE⊥=0 (blue), −35 (red) and 15 mV nm−1(green). (c)G(E⊥) atV=0. (d) Gap of layer polarizedν=2 state versusE⊥. Figure 4a plots G ( V, E ⊥ ) at ν= 2 from device 2. The most striking feature is the red region at the centre of the plot, that is, at small E ⊥ , where G~ 4 e 2 / h , surrounded by blue–white regions, where G~ 2 e 2 / h . The abrupt transition between the two regions ( Fig. 4b ) is the same as that observed in Fig. 2c . At E ⊥ =0, G ( V ) displays a narrow conductance dip at V= 0, with half-width ~1.6 mV, corresponding to Δ I ( Fig. 4c ). At large E ⊥ =−35 mV nm −1 , the G ( V ) trace is significantly different, with much wider conductance valley and half-width of 15 mV. We thus take the half-width of the wider valley to be Δ II . The dependence of Δ II on E ⊥ is shown in Fig. 4d . It increases with E ⊥ of both polarities, although with slight asymmetry. Interestingly, the wider conductance valley, which appears as the white curves superimposed on top of the blue background, extend into | E ⊥ |< E ⊥ c , that is, the narrow dip co-exists with wider valley, suggesting co-existence of both states near E ⊥ c . Figure 4: Spectroscopy data from device 2 at B =10 T and ν =2. ( a ) G ( V , E ⊥ ) data. ( b ) Line traces G ( V ) at E ⊥ =0 (blue), −35 (red) and 15 mV nm −1 (green). ( c ) G ( E ⊥ ) at V= 0. ( d ) Gap of layer polarized ν =2 state versus E ⊥ . Full size image In conclusion, we utilized high-quality dual-gated suspended BLG devices to explore the spontaneous symmetry breaking physics near charge neutrality. We resolved two distinct ν= 2 QH states: phase I is fully resolved only at E ⊥ =0 and large B , and is likely a Kekulé state with interlayer and intervalley coherence, whereas phase II is observed at small B and large E ⊥ . Our measurements demonstrate that phase II is metastable at B =0. Our data represent the first spectroscopic mapping of the exotic competing orders at ν= ±2 in BLG, and pave the way for studies of other symmetry-broken states at different filling factors in BLG or in the much less-explored TLG [8] , [53] . Our study also motivates future in-plane B measurements [9] , [54] , [55] to realize more complete control of spin, layer and orbital degrees of freedom. BLG sheets are exfoliated from Kish bulk graphite onto Si/SiO 2 substrates, and identified via colour contrast in an optical microscope and through Raman spectroscopy [56] . They are coupled to Cr (10 nm)/Au (150 nm) electrodes and Cr-suspended top gates (~300 nm above substrate) using a multi-layer lithography technique [57] , [58] , then etched in hydrofluoric acid to remove ~150–250 nm of SiO 2 . Devices are current annealed at 260 mK in He-3 refrigerators [59] , and measured using standard lock-in techniques. How to cite this article: Velasco, J. Jr et al. Competing ordered filling factor for two states in bilayer graphene. Nat. Commun. 5:4550 doi: 10.1038/ncomms5550 (2014).